Strain induced superconductivity in the parent compound BaFe2As2 The discovery of superconductivity with a transition temperature, T c , up to 65 K in single-layer FeSe (bulk T c =8 K) films grown on SrTiO 3 substrates has attracted special attention to Fe-based thin films. The high T c is a consequence of the combined effect of electron transfer from the oxygen-vacant substrate to the FeSe thin film and lattice tensile strain. Here we demonstrate the realization of superconductivity in the parent compound BaFe 2 As 2 (no bulk T c ) just by tensile lattice strain without charge doping. We investigate the interplay between strain and superconductivity in epitaxial BaFe 2 As 2 thin films on Fe-buffered MgAl 2 O 4 single crystalline substrates. The strong interfacial bonding between Fe and the FeAs sublattice increases the Fe–Fe distance due to the lattice misfit, which leads to a suppression of the antiferromagnetic spin density wave and induces superconductivity with bulk T c ≈10 K. These results highlight the role of structural changes in controlling the phase diagram of Fe-based superconductors. The discovery of Fe-based superconductors (FeSC) with critical temperatures, T c , exceeding 50 K has stimulated many experimental and theoretical efforts to reveal the mechanism for superconductivity (SC) and to find compounds with even higher T c [1] , [2] , [3] . The band structure of the stoichiometric parent compounds yields two or three small hole pockets around Γ=(0,0) and two electron pockets around M =( π , π ) in the folded zone [4] , [5] . The nesting between electron and hole bands makes the commensurate spin density wave structure (SDW) with Q =( π , π ) plausible. In all FeSCs, the transition from the paramagnetic to the magnetic-ordered SDW phase is accompanied by the structural transition from the tetragonal I 4/ mmm to the orthorhombic Fmmm phase. Doping due to injection of charge carriers (electrons or holes), chemical pressure and related disorder impairs the nesting conditions resulting in reduced structural transition temperature, T s , and Néel temperature, T N . At some finite doping, the magnetic phase gives room to SC. The vicinity to the SDW phase suggests remaining strong spin fluctuations are possibly responsible for the high-temperature SC. Therefore, the influence of doping on the phase diagram of FeSC is rather complex. Another way to realize SC in FeSC is applying external pressure [6] , [7] . Finite pressure suppresses the SDW and restores the tetragonal symmetry. As a result, SC appears with T c ’s comparable to that obtained by doping. However, the existence of SC, the value of maximum T c and the pressure under which SC occurs can vary considerably, depending on the level of hydrostaticity [8] . By investigating the pressure media with different levels of hydrostaticity, it was found that a uniaxial component of the pressure dramatically affects the phase diagram of AEFe 2 As 2 (AE122) (AE=alkali earth element) compounds [7] , [8] , [9] . It was suggested that the uniaxial pressure component is especially efficient for suppressing SDW order and responsible for a high T c of≈35 K (refs 7 , 8 , 9 ). However, to the best of our knowledge, SC under uniaxial pressure has been only reported in CaFe 2 As 2 with a relatively low T c of about 10 K (ref. 10 ). Therefore, further experimental investigations are required to clarify the relevance of uniaxial pressure for stabilizing the SC state in FeSC. In this article, we demonstrate SC in stoichiometric parent compound Ba122 thin films solely by strain. We focus on epitaxial FeSC thin films, which are currently of great interest because of the ability to modify their electronic properties solely by change of the crystal structure in a well-defined way [11] . Therefore, this method could aid understanding the conditions that can increase T c of FeSC. Recently, it was demonstrated that the bonding distances in FeAs planes might be altered by the lattice misfit to the substrate in Co-doped BaFe 2 As 2 (Ba122) [12] , [13] and in FeSe 1-x Te x (refs 14 , 15 ). As a result, variation of T c as a function of bonding distances was observed. In particular, it was discovered that SC with a transition temperature of 65 K in single-layer FeSe [16] can be induced by charge doping from the oxygen-vacant substrate to the thin film [17] (bulk T c =8 K (ref. 18 )). However, it was emphasized that the effect of strain also has an important role in driving SC [17] . To distinguish between the effects of charge doping and strain on the phase diagram of FeSC, further investigations are necessary where these two effects are decoupled. In addition, until now all the measurements regarding thin films were done for Fe-pnictide compounds that already demonstrate SC in the bulk form. In addition, we show that our data provide a deeper understanding of the mechanism responsible for controlling the phase diagram of isovalently Ru-doped Ba122. Structural analysis High-resolution reciprocal space maps ( Fig. 1a ) of the Ba122 (1 0 9) and (1 0 11 ) diffraction peaks as well as the (2 0 6) peak of the MgAl 2 O 4 (spinel) substrate reveal that substrate and thin Ba122 layers ( d ≲ d c , where d c is the critical thickness of Ba122) exhibit the same a lattice parameter ( a =0.404 nm). Increasing the thickness of the Ba122 layer to d > d c results in a relaxation of this layer, indicating a decrease of the a lattice parameter (visualized by a shift of the Ba122 diffraction peaks to larger Q x values). In the θ –2 θ scans ( Fig. 1b ), a clear trend is observed with increasing thickness, d , of Ba122. The film with d =10 nm (S 10 ) has a c lattice parameter of 1.267 nm, which is reduced by about 3% in comparison with the target value ( c =1.301 nm). For d =60 nm, two different c lattice parameters were found ( c 1 =1.279 and c 2 =1.301 nm), which is explained by partial stress relaxation within the Ba122 volume. Further increasing d results in complete stress relaxation within the whole volume of the Ba122 film. 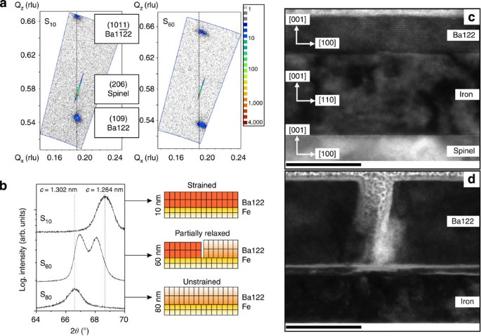Figure 1: Structural characterization by X-ray diffraction and transmission electron microscopy. (a) Reciprocal space maps of samples S10and S60. Relaxation processes for sample S60are clearly seen as a shift of the Ba122 reflections with regard to the substrate peak. The line is a guide for the eyes. (b) Evolution of the (008) diffraction peak for sample S10, S60and S80with corresponding sketches of the strain state of the Ba122 layer. The epitaxial growth of all Ba122 films was confirmed byθ–2θX-ray diffraction in the Bragg Brentano geometry and pole figure measurements (seeSupplementary Fig. S1). Bright-field TEM micrographs of two thin films: (c) sample S10(scale bar, 25 nm) and (d) sample S60(scale bar, 50 nm). The whole set of lattice constants depending on the film thickness are summarized in Table 1 . Figure 1: Structural characterization by X-ray diffraction and transmission electron microscopy. ( a ) Reciprocal space maps of samples S 10 and S 60 . Relaxation processes for sample S 60 are clearly seen as a shift of the Ba122 reflections with regard to the substrate peak. The line is a guide for the eyes. ( b ) Evolution of the (008) diffraction peak for sample S 10 , S 60 and S 80 with corresponding sketches of the strain state of the Ba122 layer. The epitaxial growth of all Ba122 films was confirmed by θ –2 θ X-ray diffraction in the Bragg Brentano geometry and pole figure measurements (see Supplementary Fig. S1 ). Bright-field TEM micrographs of two thin films: ( c ) sample S 10 (scale bar, 25 nm) and ( d ) sample S 60 (scale bar, 50 nm). Full size image Table 1 Structural and superconducting properties of the investigated samples. Full size table The mechanism of stress relaxation is also seen in bright field micrographs of sample S 10 and S 60 taken by a transmission electron microscope (TEM). The images for the beam direction parallel to the [0 1 0] direction of the spinel substrate are shown in Fig. 1c,d . The thickness of Fe and Ba122 layer for S 10 are ≈27 and 10 nm, respectively. The corresponding values for S 60 are 31 and 64 nm, respectively. In contrast to S 10 , the sample S 60 contains cracks aligned perpendicular to the film surface of Ba122 in most cases. Average distances between such cracks are in the range of a few μm and were also confirmed by atomic force microscopy (see Supplementary Fig. S2 ). Also, the root mean square roughness, R rms , was determined to be 3.5 nm for sample S 80 . This is much larger in comparison with the thinner samples ( =0.7 nm, =0.4 nm). The observed cracks are the result of the relaxation process (shortening of the a axis of the Ba122) when the critical thickness of the Ba122 layer is reached. In the vicinity of the cracks, the Ba122 layer is partially flaked from the Fe buffer layer. This leads to a formation of planar defects (probably several layers of BaO) parallel to the ab -plane as can be seen in Fig. 1d . For the films with d > d c , the observed relaxation process results in areas with properties similar to strain-free bulk Ba122 and areas that are still strained by the underlying layers (see also the sketches in Fig. 2b ). Further analysis by convergent beam electron diffraction [19] indicates that the strained state in the Ba122 layer is primarily determined by the Fe layer beneath. This is in accord with the previous observation of interfacial bonding between Fe and the FeAs sublattice of the Ba122 (ref. 20 ). 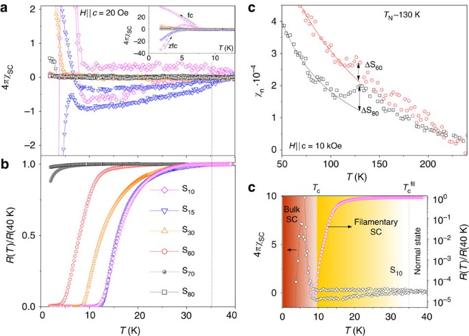Figure 2: Magnetic susceptibility and resistance. (a) Temperature dependence of the dimensionless magnetic susceptibilityχSC(T)=(m(T)−m(40 K))/VBa122Hin the superconducting state of the films with different thickness, wherem(T) is sample magnetic moment,VBa122is the volume of the Ba122 layer andHis the applied magnetic field (data are not corrected for demagnetization factors). The inset shows the region of bulk SC. (b) Temperature dependence of the normalized resistanceR(T)/R(40 K) of the investigated thin films in zero magnetic field. (c) The normal state susceptibilityχn(T)=(m(T)–m(300 K))/VBa122H. The amplitude of the SDW anomaly atTN≈130 K is reduced in the thinner film (S60), which is partially strained. (d) Susceptibility and resistance for sample S10indicating two superconducting regions (bulk SC and filamentary SC). Figure 2: Magnetic susceptibility and resistance. ( a ) Temperature dependence of the dimensionless magnetic susceptibility χ SC (T)=( m ( T )− m (40 K))/ V Ba122 H in the superconducting state of the films with different thickness, where m ( T ) is sample magnetic moment, V Ba122 is the volume of the Ba122 layer and H is the applied magnetic field (data are not corrected for demagnetization factors). The inset shows the region of bulk SC. ( b ) Temperature dependence of the normalized resistance R ( T )/ R (40 K) of the investigated thin films in zero magnetic field. ( c ) The normal state susceptibility χ n ( T )=( m ( T )– m (300 K))/ V Ba122 H . The amplitude of the SDW anomaly at T N ≈130 K is reduced in the thinner film (S 60 ), which is partially strained. ( d ) Susceptibility and resistance for sample S 10 indicating two superconducting regions (bulk SC and filamentary SC). Full size image Magnetic properties The SC properties of the films were investigated using several complementary techniques. The temperature dependence of the dimensionless volume magnetic susceptibility χ SC ( T )=( m ( T )− m (40 K))/ V Ba122 H and the normalized resistance R ( T )/ R (40 K) for films with various thickness are shown in Fig. 2 , where m ( T ) is the sample magnetic moment, V Ba122 is the volume of the Ba122 layer and H is the applied magnetic field. A decrease of d results in an increase of the superconducting T c and the SC volume fraction of the films. The upturn of the susceptibility in the SC state is probably caused by the paramagnetic Meissner effect (Wohlleben effect) [21] , [22] , [23] , [24] . The large value of the diamagnetic signal at low temperatures suggests that an essential volume of the films is in the SC state at low T (see inset of Fig. 2a ). The temperature dependence of the normal volume magnetic susceptibility χ n ( T )=( m ( T )− m (300 K))/ V Ba122 H for films S 80 and S 60 is shown in Fig. 2c . As can be seen, the amplitude of the SDW anomaly at T N ~130 K is reduced in the thinner film (S 60 ), which is partially strained. Moreover, no signature of the SDW transition was observed for the films with d <60 nm, suggesting that in-plane tensile strain effectively suppresses long-range SDW order and SC does not coexist with SDW order in the thin films. T N ~130 K of the unstrained thick films is consistent with T N ≈140 K observed in stoichiometric BaFe 2 As 2 single crystals [25] . Electrical transport properties The SC transition width, Δ T c = T c,onset − T c , of the films is very large ( Fig. 2b,d ). For films with d <30 nm, the decrease of resistance starts at relatively high temperatures T c,onset = ≈35 K, whereas zero resistance is measured at T c ≈10 K as shown in Fig. 2c,d . As can be seen in Fig. 2d , exactly corresponds to the temperature at which splitting between zero field-cooled and field-cooled branches of the susceptibility χ ( T ) curves is observed. In turn, a strong signal in susceptibility data for the thin films with d <30 nm is observed below T c only ( Fig. 2a ). From the ratio between diamagnetic moments at T >10 K and in the low- T region, we concluded that in the range between and T c ≈10 K, SC exists only in a small volume fraction of the films. This so-called filamentary SC [7] , [26] (see Supplementary Fig. S3 ) is attributed to minor regions with slightly different strain state. The values of T c and , given in Table 1 and Fig. 4, are deduced from the method presented in Fig. 2d . Critical current densities The presence of the ferromagnetic Fe buffer layer and the extremely planar geometry of the films (large demagnetization factor) do not allow to estimate directly the SC volume fraction from the diamagnetic screening at low temperatures (see Fig. 2a ). Therefore, we additionally measured the transport critical current density, J c , to demonstrate that a large volume of the films is in the superconducting state below T c . It is seen in Fig. 3a that self-field J c values in the strained film S 30 are comparable to the ones in optimally Co-doped Ba122 epitaxial thin films having a similar thickness d ≈30 nm and T c ≈22 K (ref. 27 ) We suppose that the different J c and irreversibility field for sample S 30 and sample S 10 are due to different pinning properties rather than related to grain connectivity or other extrinsic factors. A dominant weak-link behaviour is excluded by the relative robustness of J c to external magnetic fields (see Fig. 3b,c ). Moreover, we exclude a large variation of the cross-section for the superconducting currents as we observed a comparable diamagnetic signal for both films (see Fig. 2a ). Thus, the relatively high J c values obtained from transport current measurements are an additional strong evidence for a large SC volume of the films with d ≤30 nm. 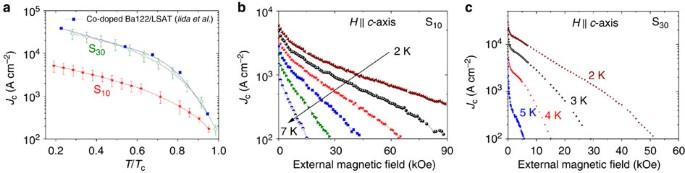Figure 3: Critical current densities. (a) Temperature dependence of self-fieldJcfor sample S10and S30compared with data on Co-doped Ba122 taken from ref.27. The relatively largeJcvalues indicate bulk SC for the strained films. BulkTc,0was taken for normalizing the data. The error bars are caused by the uncertainty in the film thickness due to the surface roughness (minimal and maximal size of Ba122 layer thickness). (b) and (c) provideJc(B) data for samples S10and S30, respectively. Figure 3: Critical current densities. ( a ) Temperature dependence of self-field J c for sample S 10 and S 30 compared with data on Co-doped Ba122 taken from ref. 27 . The relatively large J c values indicate bulk SC for the strained films. Bulk T c,0 was taken for normalizing the data. The error bars are caused by the uncertainty in the film thickness due to the surface roughness (minimal and maximal size of Ba122 layer thickness). ( b ) and ( c ) provide J c ( B ) data for samples S 10 and S 30 , respectively. Full size image We suppose that the main mechanism of inducing SC and, therefore, controlling the phase diagram of Ba122 in our films is tensile in-plane strain. To investigate the possible role of charge transfer from the Fe buffer to the Ba122 layer similar to the case of FeSe single layers (see Introduction), we compared the strained films with a non-strained one grown on different substrates but having similar thickness of Ba122 and Fe-buffer layers. It was found that the unstrained films do not show any signature of a superconducting transition (see Supplementary Fig. S4 ). Thus, a sizable effect of the proximity to the metallic Fe buffer layer on T c is ruled out. We sum up our main findings in Fig. 4 and Table 1 . As can be seen, the films with thickness d < d c ≈30 nm having a large SC volume fraction are completely strained. The Ba122 layer relaxes and the SC volume abruptly reduces when the thickness exceeds d c . The films with d ~80 nm have lattice parameters as unstrained bulk Ba122 and a negligibly small SC volume fraction. To gain a deeper understanding of the relevant parameters for tuning the Ba122 phase diagram, we compare our results with data of isovalently Ru-doped Ba122 (refs 25 , 28 ). As can be seen in Table 1 , the lattice parameters and T c values of overdoped Ba(Fe 1− x Ru x ) 2 As 2 with x ~0.4−0.5 are comparable to the values of our thin films. These striking similarities evidence that structural changes induced by Ru doping are the dominant factor in controlling the phase diagram. Other factors that were assumed to explain the emergence of SC in Ru-doped Ba122 (disorder effects, dilution of the magnetic Fe sublattice and an enhancement in the bandwidth due to hybridization involving Ru [29] , [30] ), only have a secondary role. From this point of view, disorder may explain the variations of T c and the shifting of the SC dome in the phase diagram for different samples of Ru-doped Ba122 (refs 25 , 28 , 31 ). Moreover, the comparison between our data on strained Ba122 and the phase diagram of Ru-doped single crystals together with the observed mechanism of stress relaxation (as discussed above) shed a light on the filamentary SC with ≈35 K found in the thinnest films (see Fig. 3 ). The SC regions with can be related to minor regions with reduced strain (most probably because of low-angle grain boundaries) of the Ba122 layer. Therefore, these regions have slightly smaller a and larger c lattice parameters compared with the main strained phase, which is consistent with an analysis using electron backscatter diffraction (Chekhonin P. et al. , unpublished). In particular, this shows that T c ≥35 K is possible by adjusting the lattice strain of Ba122. 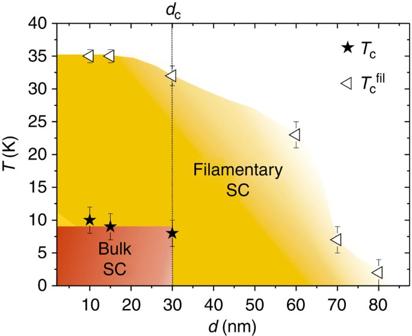Figure 4: SchematicTc−ddiagram for parent compound BaFe2As2thin films. Filled symbols denoteTcof the main superconducting phase. Open symbols show onsetof the filamentary SC. Fordc>30 nm the SDW transition was observed atTN~130 K. The colours are guide for the eyes. The error bars were estimated by the s.d. of magnetic and transport measurement data. Figure 4: Schematic T c − d diagram for parent compound BaFe 2 As 2 thin films. Filled symbols denote T c of the main superconducting phase. Open symbols show onset of the filamentary SC. For d c >30 nm the SDW transition was observed at T N ~130 K. The colours are guide for the eyes. The error bars were estimated by the s.d. of magnetic and transport measurement data. Full size image Finally, we conclude that the coherent interfacial bonding between Fe and the FeAs sublattice of the Ba122 results in an in-plane straining of Ba122 to the (001) plane of bcc Fe-buffer layer, that is, increasing a and reducing c lattice parameters of the Ba122 layer for thicknesses d < d c ≈30 nm. This suppresses magnetism and gives rise to bulk SC with T c ≈10 K. The large superconducting volume fraction of the films with d ≤ d c is evidenced by a pronounced diamagnetic screening and by measurements of a finite transport critical current. The close similarities of crystal parameters and T c between thin films and Ru-doped Ba122 indicate that structural changes are one of the dominant factors for controlling T c of Ba122. Further, the observation of filamentary SC at 35 K in regions with a different strain state suggests that T c 35 K is possible in Ba122 without doping or applying external pressure. Sample preparation The targets used for the thin film growth were prepared by a conventional solid state reaction process as described in refs 12 , 13 , 33 . The thin films were grown using pulsed laser deposition with a KrF excimer laser ( λ =248 nm). The preparation process took place in an ultra-high vacuum chamber with a base pressure of 10 −9 mbar. Before the deposition, the substrate was heated up to 750 °C to clean the surface. Subsequently, the Fe buffer layer of about 30 nm thickness was deposited at room temperature with a laser frequency of 5 Hz and then heated to 670 °C to flatten the Fe surface [20] , [32] . This temperature was held for 30 min before the Ba122 layer was grown with a frequency of 10 Hz. The layer thickness was adjusted via the pulse number at constant laser energy and was confirmed by TEM for selected samples. To achieve homogeneous samples without thickness gradient, the substrate was rotated during the whole deposition. Structural characterization The c lattice parameters were calculated from X-ray diffractograms (in a Bruker D8 Advance Diffraktometer) in Bragg Brentano geometry using the Nelson Riley function, whereas the a lattice parameters were taken out of the reciprocal space maps measured in a Panalytical X’pert Pro system. TEM characterization of the samples was performed at FEI Tecnai-T20 TEM operating at an accelerating voltage of 200 kV. Preparation of the TEM lamellae was done by the focused ion beam technique (FEI Helios 600i) using a platinum protection layer and 3 kV accelerating voltage in the last focused ion beam preparation step. Electron diffraction X-ray spectroscopy in TEM and auger electron spectroscopy were performed to check the Ba122 stoichiometry. Sensitivity factors for the auger electron spectroscopy spectra were evaluated using single crystals [33] . Parts of the thin film and the single crystal were sputtered, and the resulting spectra were analysed in a JEOL JAMP 9500F field emission Auger microprobe (see Supplementary Fig. S5 ). The resulting data are given in supplement and confirm that the thin films are stoichiometric. Transport and magnetic measurements Transport measurements were performed using a physical property measurement system (Quantum Design) with four probe method. Magnetic measurements were performed in a Quantum Design direct current superconducting quantum interference device. In the normal state, electrical currents flow mainly through the metallic Fe buffer layer having a lower resistance than the Ba122 layer. Hence, it is not possible to measure the SDW/structural transition via transport measurements. For the measurements of the critical current density, J c , the samples S 10 and S 30 were structured using ion beam etching with a stainless steel mask. Bridges of 0.45 mm width and 0.6 mm length were fabricated. J c was determined from E ( J ) characteristics using the geometry parameters of the bridges and applying a 1 μV cm −1 criterion ( J ⊥ H —max. Lorentz force configuration). How to cite this article: Engelmann, J. et al. Strain induced superconductivity in the parent compound BaFe 2 As 2 . Nat. Commun. 4:2877 doi: 10.1038/ncomms3877 (2013).